Contrasting arbuscular mycorrhizal responses of vascular and non-vascular plants to a simulated Palaeozoic CO2decline The arbuscular mycorrhizal (AM) fungal symbiosis is widely hypothesized to have promoted the evolution of land plants from rootless gametophytes to rooted sporophytes during the mid-Palaeozoic (480–360 Myr, ago), at a time coincident with a 90% fall in the atmospheric CO 2 concentration ([CO 2 ] a ). Here we show using standardized dual isotopic tracers ( 14 C and 33 P) that AM symbiosis efficiency (defined as plant P gain per unit of C invested into fungi) of liverwort gametophytes declines, but increases in the sporophytes of vascular plants (ferns and angiosperms), at 440 p.p.m. compared with 1,500 p.p.m. [CO 2 ] a . These contrasting responses are associated with larger AM hyphal networks, and structural advances in vascular plant water-conducting systems, promoting P transport that enhances AM efficiency at 440 p.p.m. [CO 2 ] a . Our results suggest that non-vascular land plants not only faced intense competition for light, as vascular land floras grew taller in the Palaeozoic, but also markedly reduced efficiency and total capture of P as [CO 2 ] a fell. Arbuscular mycorrhizal (AM) fungi are among the most ancient and widespread obligate symbionts in contemporary floras, and are dependent on host plants for carbon, as they lack saprotrophic capabilities [1] . AM fungi are highly adapted to mobilize and translocate phosphorus (P) from beyond root depletion zones and from pores too small for entry by root hairs, in return for receiving photosynthate carbon [1] . Physiological adaptations include phosphate transporters within hyphal membranes with very high affinities for soil P, and phosphate transporters located in arbuscules that transfer P from the fungus to the plant cortex cells [2] . Phylogenetic relationships of mycorrhiza-specific genes coding for AM-inducible plant P transporters indicate their involvement in symbiotic P transport for hundreds of millions of years, with highly conserved regulation of gene expression [2] . The basis of the AM mutualism involves a stable cooperation between partners. Host plants preferentially reward fungal partners that provide greater access to P with photosynthate, and the fungi allocate P preferentially to plant partners providing a greater carbohydrate supply [3] . Phosphorus is an essential element required by plants for core metabolism (ATP) and growth (phospholipid membranes, RNA and DNA), and its low availability in soils is often a primary constraint on the productivity of terrestrial ecosystems [4] . This requirement has driven the establishment of symbiotic partnerships between soil-dwelling fungi and the earliest land plants (embryophytes) to increase the uptake of P ever since plants' initial conquest of the land [5] , [6] , [7] . Intercellular hyphae and arbuscules have been documented in gametophytes and sporophytes from the Early Devonian Rhynie chert flora, together with exceptionally well-preserved spores representative of several of the major glomeralean fungal groups [8] , [9] , [10] , [11] , [12] . These associations with AM fungi formed under a CO 2 -rich atmosphere, even before true roots evolved around 400 Myr, ago ( Fig. 1 ). 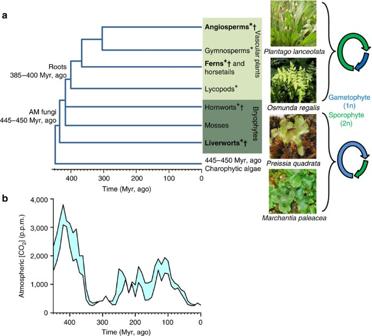Figure 1: Co-evolution of land plant lifecycles and atmospheric CO2concentrations. (a) depicts land plant phylogeny (adapted from (refs.47,48) and (b) the modelled global [CO2]ahistory (adapted from (ref.24)) for the past 500 Myr, ago. Mapped onto the phylogeny is the occurrence of AM fungal associations across plant taxa*, and fossil evidence of AM fungi†. Species investigated in this work are highlighted in bold and pictured right. Dominant stages of plant life cycles are shown as 1n(gametophyte) and 2n(sporophyte). Figure 1: Co-evolution of land plant lifecycles and atmospheric CO 2 concentrations. ( a ) depicts land plant phylogeny (adapted from (refs. 47 , 48 ) and ( b ) the modelled global [CO 2 ] a history (adapted from (ref. 24 )) for the past 500 Myr, ago. Mapped onto the phylogeny is the occurrence of AM fungal associations across plant taxa * , and fossil evidence of AM fungi † . Species investigated in this work are highlighted in bold and pictured right. Dominant stages of plant life cycles are shown as 1 n (gametophyte) and 2 n (sporophyte). Full size image The subsequent diversification of embryophytes in the mid-Palaeozoic (480–360 Myr, ago) is marked by the transition from a gametophyte-dominant generation lifecycle to one with an increasingly elaborate sporophyte-dominant generation, and the evolutionary appearance of roots, leaves and other innovations [13] . As terrestrial plants and ecosystems evolved, they progressively grew in stature, biomass, nutrient demand and rooting depth to extensively colonize uplifted continental land masses. The resulting increase in below-ground export of photosynthate carbon energy drove enhanced silicate rock weathering [14] , the development of soil profiles, pedogenic clay minerals [15] , [16] , [17] and organic carbon burial [18] , [19] . Enhanced biological weathering from 410–340 Myr, ago is linked to a 90% reduction in the atmospheric CO 2 concentration ([CO 2 ] a ) through the release of Ca and Mg from silicate minerals, and their export to the oceans where they were precipitated into carbonate sediments ( Fig. 1 ) [18] , [20] . During the mid Palaeozoic, co-evolution of the AM fungal symbiosis and rooting systems likely had a pivotal role in provisioning the expanding biomass, stature and biogeography of forested ecosystems with their rising demand for essential soil nutrients. This would be especially important as P became increasingly limited owing to depletion of the primary mineral apatite (calcium phosphate) by chemical and biological weathering [4] , [21] ( Fig. 1 ). Here we investigate the hypothesis that the evolutionary transition from non-vascular to vascular embryophytes with sporophyte-dominant lifecycles as Palaeozoic [CO 2 ] a declined, drove changes in the plant–fungal cost benefits of the AM symbiosis. Our approach is based on the development and application of dual 33 P and 14 C isotope tracers to measure the reciprocal fluxes of carbon from plant-to-fungus, and phosphorus from fungus-to-plant. These fluxes are quantified using mesh-walled cores filled with soil set around the plants that can be colonized by AM hyphae but not plant roots or rhizoids. Static cores preserve intact hyphal networks running into the core, whereas rotated cores severe the network. AM symbiosis efficiency is defined as P gained by the plant through its fungal partners per unit of photosynthate carbon invested into the P absorbing hyphal network in the undisturbed mesh cores. This novel metric allows AM symbiosis efficiency to be determined for whole plants growing in natural soil, and facilitates comparisons across taxa and environments. Experiments were conducted with plant species representing three key nodes on the land plant evolutionary tree spanning several hundred million years of terrestrial ecosystem evolution ( Fig. 1 ). These nodes encompass the critical transition from non-vascular plant gametophyte-dominant to vascular plant sporophyte-dominant lifecycles and appearance of true roots [13] . We investigated two species of basal non-vascular land plants (complex thalloid liverworts) with rhizoid systems ( Preissia quadrata and Marchantia paleacea ), grown either as prostrate mats of gametophytes ( P. quadrata ), or as individual gametophytes ( M. paleacea ). Both species of liverworts belong to the phylogenetic sub-group of Marchantiopsida [22] . Liverwort gametophyte [CO 2 ] a responses were compared with those of the sporophytes of the basal vascular land plant Osmunda regalis , a fern with a well-developed rooting system, and the advanced angiosperm Plantago lanceolata , which has a coarse rooting system and high mycorrhizal dependency. 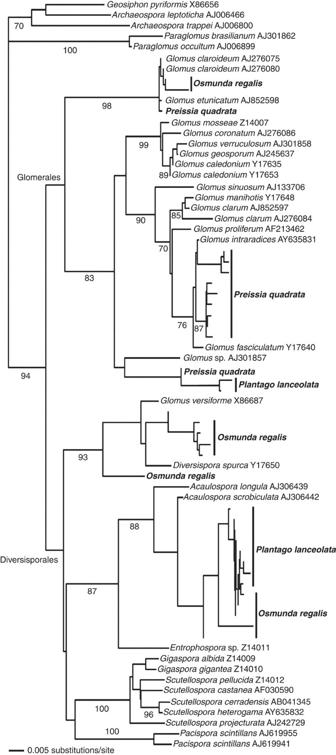Figure 2: Molecular identification of plant–AM-fungal symbionts. Neighbour-joining distance tree of fungi based on 960 bp of 5′ 18S nuclear ribosomal DNA sequences. Bootstrap percentages are shown below branches. Plant species names are given in bold. DNA sequencing of the fungal partners within host root/thallus samples of our experimental plants confirmed they formed associations with AM fungi of the Glomeromycota ( Fig 2 ). Plants were grown on skeletal nutrient-poor dune soil approximating the oligotrophic conditions of Palaeozoic terrestrial environments [23] and at 1,500 p.p.m. and 440 p.p.m. [CO 2 ] a as values representative of mid- and late-Palaeozoic atmospheres, respectively ( Fig. 1 ) [24] . We found that AM symbiosis efficiency responds differently to a simulated Palaeozoic [CO 2 ] a decline from 1,500 p.p.m. to 440 p.p.m. ; decreasing in the most basal non-vascular land plant group (liverworts) and increasing in two vascular groups (ferns and angiosperms). These contrasting responses are associated with the structural advances in vascular plant water-conducting systems in roots and shoots enhancing physiological feedbacks that promote P translocation through the fungus and overall AM efficiency at 440 p.p.m. [CO 2 ] a . Our experiments provide new insight into how the evolutionary advance from root-less gametophytes to rooted sporophytes increased the efficiency of biogeochemical cycling of P in soils during the 'greening of the Earth'. Figure 2: Molecular identification of plant–AM-fungal symbionts. Neighbour-joining distance tree of fungi based on 960 bp of 5′ 18S nuclear ribosomal DNA sequences. Bootstrap percentages are shown below branches. Plant species names are given in bold. Full size image Plant and fungal C-fluxes respond to [CO 2 ] a treatments Over the 4-month duration of the experiments, the above-ground biomass of fern sporophytes was significantly (two-way ANOVA, F 3,23 =3.31, P <0.05) lower by 50% at 440 p.p.m. compared with 1,500 p.p.m. [CO 2 ] a , whereas the Preissia and Marchantia gametophytes, and the angiosperm sporophytes, showed no significant response to CO 2 (two-way ANOVA, F 3,23 =3.31, P >0.05) ( Fig. 3a ). These biomass differences are linked to changes in plant carbon allocation to AM fungal networks inside the mesh-walled soil cores. One liverwort species, and both vascular plant species, exhibited significantly (two-way ANOVA, F 3,23 =40.18, P <0.05) lower (by over 90%) carbon allocation to the AM fungal networks colonizing the soil cores when grown at 440 p.p.m. compared with 1,500 p.p.m. [CO 2 ] a , as traced by 14 CO 2 supplied to the shoots ( Fig. 3b ). Plant carbon allocation to fungi therefore seems to be a [CO 2 ] a -sensitive component of the AM symbiosis. Despite this reduced carbon investment in the AM networks, both liverworts and the fern pay a higher cost to support them at 440 p.p.m. [CO 2 ] a , when calculated as the percentage 14 CO 2 fixed over a 12-h photoperiod ( Fig. 3c ). 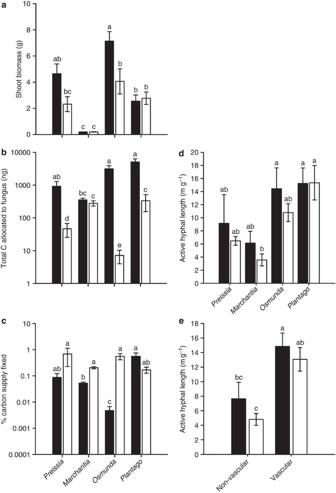Figure 3: Plant and fungal responses to [CO2]atreatments. Responses of (a) above-ground tissue biomass, (b) total carbon allocation to fungus within soil cores, (c) the percentage of total plant-fixed carbon allocated to fungus within soil cores, (d) the active hyphal length of fungi within soil cores and (e) active hyphal lengths in soil cores for the non-vascular and vascular plant species grown at 1,500 p.p.m. (black bars) or 440 p.p.m (white bars) [CO2]a. Bars with no letters in common are significantly different atP<0.05 (Tukey test after two-way ANOVA with species and [CO2]aand their interaction), whereas those sharing the same letters are not statistically significantly differentP>0.05). Two-way ANOVA detected significant (P<0.01) effects of plant species in (a–d), and [CO2]atreatments in (a), (b) and (d) (P<0.05). Species×[CO2]atreatment interactions are significant in (a) and (b) (P<0.05), but not (c) and (d) (P>0.5). In all panels, means are shown ±1 s.e.m. (n=4). Figure 3: Plant and fungal responses to [CO 2 ] a treatments. Responses of ( a ) above-ground tissue biomass, ( b ) total carbon allocation to fungus within soil cores, ( c ) the percentage of total plant-fixed carbon allocated to fungus within soil cores, ( d ) the active hyphal length of fungi within soil cores and ( e ) active hyphal lengths in soil cores for the non-vascular and vascular plant species grown at 1,500 p.p.m. (black bars) or 440 p.p.m (white bars) [CO 2 ] a . Bars with no letters in common are significantly different at P <0.05 (Tukey test after two-way ANOVA with species and [CO 2 ] a and their interaction), whereas those sharing the same letters are not statistically significantly different P >0.05). Two-way ANOVA detected significant ( P <0.01) effects of plant species in ( a – d ), and [CO 2 ] a treatments in ( a ), ( b ) and ( d ) ( P <0.05). Species×[CO 2 ] a treatment interactions are significant in ( a ) and ( b ) ( P <0.05), but not ( c ) and ( d ) ( P >0.5). In all panels, means are shown ±1 s.e.m. ( n =4). Full size image Because AM fungi are obligate biotrophs dependent on their host plants for photosynthate energy [1] , we next determined how patterns of plant C allocation translated into changes in the size of the active nutrient-absorbing fungal network. Active mycorrhizal networks in soil cores were estimated as the difference in hyphal lengths per unit mass of soil between the static and rotated mesh cores. In general, changes in the size of active fungal lengths were less responsive to the two [CO 2 ] a treatments than C allocation ( Fig. 3d ). Such modest [CO 2 ] a effects on hyphal lengths may be due to persistence of severed hyphae in the rotated cores for which turnover times are uncertain and extremely difficult to determine [25] . In addition, although our estimates of the active hyphal network predominantly reflect changes in populations of mycorrhizal fungi, there will be a saprotrophic fungal component, which may partially obscure responses exclusively attributable to AM hyphae. At the individual species–level, there was no significant (two-way ANOVA, F 1,23 =0.24, P > 0.05) effect of [CO 2 ] a on active hyphal lengths, although there was a consistent trend for lower values in both liverwort species and the fern ( Fig. 3d ). However, pooling the data for each of the two types of plant (that is, non-vascular and vascular), revealed that the liverworts supported active hyphal lengths that were significantly (by 48%) smaller than those of the vascular plants at 1,500 p.p.m., and 63% lower at 440 p.p.m. [CO 2 ] a (two-way ANOVA, F 1,24 =17.80, P <0.05 in both cases) ( Fig. 3e ). This finding is in keeping with the small size, prostrate habit, low productivity and absence of roots in the liverworts. Fungal 33 P uptake responds to [CO 2 ] a treatments We next examined the functionality of the fungal hyphal networks in the soil cores, as determined by their uptake and delivery of 33 P from the cores to the plants ( Fig. 4 ). Tissue concentrations of 33 P ( Fig. 4a ) indicate that the sporophytes of both vascular plant taxa (fern and angiosperm) maintained fungal-acquired 33 P uptake at 1,500 p.p.m. and 440 p.p.m. [CO 2 ] a , despite significant (two-way ANOVA, F 3,23 =52.04, P <0.05) reductions in carbon allocation to the fungi inside the soil cores at the lower [CO 2 ] a ( Fig. 3b ). In contrast, gametophytes of the liverwort P. quadrata showed dramatically lower (3–4 orders of magnitude) 33 P uptake when grown at 440 p.p.m. compared with 1,500 p.p.m. [CO 2 ] a ( Fig. 4a,b ), linked to the reduced carbon investment into fungal mycelia ( Fig. 3b ). Similarly the second liverwort species, M. paleacea , also showed a significant (two-way ANOVA, F 3,23 =48.06, P <0.05) near 10-fold reduction in 33 P uptake at 440 p.p.m. compared with 1,500 p.p.m. [CO 2 ] a . 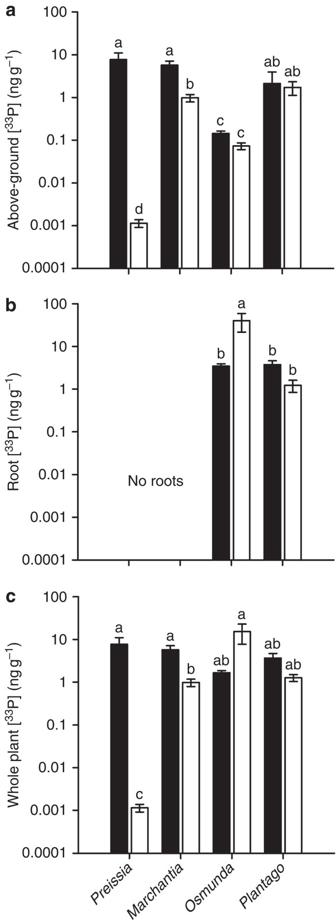Figure 4: Uptake of33P by hyphal networks in response to [CO2]atreatments. Mean total33P concentrations (ng g−1) in (a) above-ground tissues, (b) below-ground tissues and (c) within whole plants for each species at 1,500 p.p.m. (black bars) or 440 p.p.m. (white bars□) [CO2]a. Bars with no letters in common are significantly different atP<0.05 (Tukey test after two-way ANOVA with species and [CO2]aand their interaction), whereas those sharing the same letters are not statistically significantly differentP>0.05). Two-way ANOVA detected significant (P<0.05) effects of plant species in (a–c), and [CO2]atreatments (P<0.001) in (a) and (c). Species×[CO2]atreatment interactions are significant in (a), (b) and (c) (P<0.01). In all panels, means are shown ±1 s.e.m. (n=4). Figure 4: Uptake of 33 P by hyphal networks in response to [CO 2 ] a treatments. Mean total 33 P concentrations (ng g −1 ) in ( a ) above-ground tissues, ( b ) below-ground tissues and ( c ) within whole plants for each species at 1,500 p.p.m. (black bars) or 440 p.p.m. (white bars□) [CO 2 ] a . Bars with no letters in common are significantly different at P <0.05 (Tukey test after two-way ANOVA with species and [CO 2 ] a and their interaction), whereas those sharing the same letters are not statistically significantly different P >0.05). Two-way ANOVA detected significant ( P <0.05) effects of plant species in ( a – c ), and [CO 2 ] a treatments ( P <0.001) in ( a ) and ( c ). Species×[CO 2 ] a treatment interactions are significant in ( a ), ( b ) and ( c ) ( P <0.01). In all panels, means are shown ±1 s.e.m. ( n =4). Full size image When comparing differences in P concentrations between taxa, it is important to recognize that the fern and angiosperm shoots are free of mycorrhizal fungi, whereas liverwort gametophyte thalli include fungal-colonized cells, which may retain 33 P not transferred to the plant. To ensure comparability across taxa, therefore, we also calculated whole plant 33 P concentrations by including its concentration in roots, where present, which can also retain 33 P either in plant or fungal tissues ( Fig. 4b ). Calculated on this basis, the results support the finding that neither of the two vascular plant species showed significant reductions (two-way ANOVA, F 3,23 =69.02, P <0.05: Tukey multiple comparison between species and CO 2 P > 0.05) in 33 P uptake at the lower growth [CO 2 ] a , whereas it fell significantly (two-way ANOVA, F 3,23 =69.02, P <0.05) in both liverwort taxa ( Fig. 4c ). AM symbiosis efficiency responds to [CO 2 ] a treatments We quantified the functional efficiency of the AM symbiosis based on the 14 C and 33 P tracer results, defined as total 33 P taken up from the mesh-walled soil cores and transported into above-ground tissues ( Fig. 4 ) per unit of photosynthate allocated to the AM fungal hyphae within these cores ( Fig. 3 ), denoted as shoot 33 P/C ( Fig. 5 ). Calculated on this basis, there were strong differential responses of 33 P/C AM efficiency to the two [CO 2 ] a values with the evolution of plant lifecycles. Liverwort gametophytes exhibited 10- to 100-fold reductions in AM symbiosis efficiency at 440 p.p.m. compared with 1,500 p.p.m. [CO 2 ] a , which was significant (two-way ANOVA, F 3,23 =46.16, P <0.05) in Preissia , whereas both vascular plant taxa showed significant (two-way ANOVA, F 3,23 =46.16, P <0.05) 10- to 100-fold increases ( Fig. 5 ). 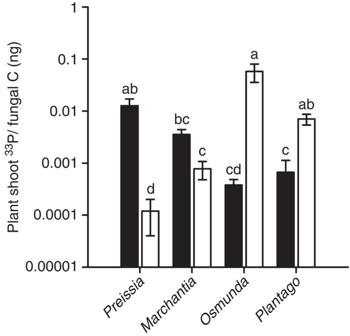Figure 5: Response of AM symbiosis efficiency to [CO2]atreatments. Plant AM symbiosis efficiency measured as phosphorus-for-carbon efficiency (total P (ng)/total C(ng)) at 1,500 p.p.m. (black bars) or 440 p.p.m. (white bars□) [CO2]a. Bars sharing the same letters are not statistically significantly different (Tukey test after two-way ANOVA (species and [CO2]atreatments)P>0.05), whereas those with no letters in common are different atP<0.05. Two-way ANOVA detected significant effects of plant species (P<0.05), but not [CO2]atreatments (P=0.85). Species×[CO2]atreatment interaction is significant (P<0.001). In all panels, means are shown ±1 s.e.m (n=4). Figure 5: Response of AM symbiosis efficiency to [CO 2 ] a treatments. Plant AM symbiosis efficiency measured as phosphorus-for-carbon efficiency (total P (ng)/total C(ng)) at 1,500 p.p.m. (black bars) or 440 p.p.m. (white bars□) [CO 2 ] a . Bars sharing the same letters are not statistically significantly different (Tukey test after two-way ANOVA (species and [CO 2 ] a treatments) P >0.05), whereas those with no letters in common are different at P <0.05. Two-way ANOVA detected significant effects of plant species ( P <0.05), but not [CO 2 ] a treatments ( P =0.85). Species×[CO 2 ] a treatment interaction is significant ( P <0.001). In all panels, means are shown ±1 s.e.m ( n= 4). Full size image Extant liverworts are descended from embryophytes that diverged before tracheophytes appeared [26] . Comparative experiments between liverworts and tracheophyte lineages therefore provide a unique window into the physiological processes behind the early evolution of land plants. Under the high [CO 2 ] a prevailing during the early stages of embryophyte colonization of the land [24] , gametophytes of two species of the basal non-vascular plant group (liverworts) operated with the highest AM symbiosis efficiency of all extant taxa investigated ( Fig. 5 ). It effectively amplified the benefits of the AM symbiosis to these non-vascular 'lower' plants by reducing the carbon cost of fungal-acquired P from the soil ( Fig. 5 ). Recent studies established that high [CO 2 ] a and AM fungal colonization synergistically enhance the photosynthetic capacity, growth and reproductive fitness of liverworts [6] . Our new measurements of AM symbiosis efficiency provide further support reinforcing the hypothesis that the high [CO 2 ] a of the early Palaeozoic created a strong selection pressure favouring the establishment of mycorrhiza-like partnerships with AM fungi in the gametophyte-dominant phase of rootless early land plants [6] , [8] , [27] . Our experimental findings suggest that the dramatic fall in [CO 2 ] a through the mid-Palaeozoic penalized the AM efficiency of non-vascular liverwort gametophytes, but enhanced it in more evolutionarily advanced vascular plant sporophytes. The differential nature of this AM symbiosis efficiency response across plant taxa quantified here ( Fig. 5 ) is linked to the relative insensitivity of vascular plant 33 P uptake via AM fungi between 1,500 and 440 p.p.m. [CO 2 ] a and its sensitivity in liverworts ( Fig. 4 ). This is associated with the large (14.8 m g −1 ) AM hyphal networks associated with the vascular plants showing little response to [CO 2 ] a . However, the AM networks of liverworts, which were only half the length of those of the vascular plants (7.7 m g −1 ) at 1,500 p.p.m., showed a proportionally greater decline of 38% at 440 p.p.m. [CO 2 ] a , although this was not significant (two-way ANOVA, F 1,24 =0.908, P >0.05) owing to high variance between replicates. Fungal P uptake kinetics are linked to hyphal network size. Both experimental evidence [28] , [29] , [30] and theory [31] indicate that inorganic P uptake by AM fungi follows Michaelis–Menton saturation kinetics, approaching an asymptote, as hyphal density in the soil increases. Further reductions in hyphal lengths from already low values in liverworts therefore result in very large declines in P uptake, not seen in the vascular plants with larger networks [30] . Transpiration rates of leaves, and the translocation of P through fungal hyphae, are strongly linked to the mass flow of nutrients into the plants, increasing the effective region of P uptake around hyphae [32] . For example, maximum rates of transpiration of the herbaceous angiosperm Trifolium repens grown in association with the AM fungus Glomus mosseae increased total P translocation by the fungus to the host by >2-fold compared with plants with low transpiration rates [32] . Such plant physiological feedbacks operate, in part, by promoting replenishment of the immediate depletion zones around the AM hyphae, and reducing the energetic costs of active transport of P to the plant by cytoplasmic streaming through the fungal network [1] . In vascular plants from across a wide phylogenetic spectrum (including clubmosses, ferns and angiosperms), leaf stomatal size and density, and the resulting operational stomatal conductance to water vapour, are higher at 440 p.p.m. than at 1,500 p.p.m. [CO 2 ] a [33] . This plasticity in vascular plant responses to lower [CO 2 ] a , together with advances in water-conducting tissues, causes their transpiration rates to increase raising the efficiency of their AM hyphal networks. In contrast, the anatomically simpler liverworts, which grow appressed to their moist substrate, and lack the plasticity of tissue porosity in response to changing [CO 2 ] a , have no apparent means of increasing the mass flow of nutrients into their thallus as [CO 2 ] a falls. In the context of the dramatic evolutionary changes that occurred in plants through the Palaeozoic [CO 2 ] a decline [13] , these physiological effects promoting AM efficiency by enhancing soil P uptake, without requiring additional host plant C investment in fungi, were likely to be strongly reinforced. Major evolutionary innovations appeared including vascular tissues, progressively larger leaves with increasingly numerous stomata [34] , [35] , and deeper rooting systems [36] , [37] enabling greater canopy transpiration and mass flow of nutrients from the soil solution into plants. By increasing mass transport of nutrients into roots with an expanding plant biomass, these innovations likely generated positive plant physiological feedback mechanisms progressively enhancing AM symbiosis efficiency by reducing the carbon cost to the host plants per unit of nutrient supplied via mycorrhiza. Such mechanisms are clearly not applicable to the ancestral and structurally simple gametophytes of early non-vascular land plants lacking both stomata and roots. As burgeoning terrestrial floras began consuming the immediately accessible supplies of P on land making it increasingly scarce, they created strong selection pressures for more efficient plant–fungal AM symbiosis with a fall in Palaeozoic [CO 2 ] a . Indeed, recent studies have highlighted a consistent property of ecosystem development over tens of thousands to millions of years is decreasing P availability, as it becomes locked up in recalcitrant secondary minerals and organic matter, and depleted via weathering, erosion and leaching [21] . Overall, these results imply that non-vascular land plants faced not only intense competition for light, as the evolving vascular land floras grew taller in the Palaeozoic [13] , [38] but also experienced a greatly reduced efficiency and total capture of P with the fall in [CO 2 ] a . We conclude that increasing mycorrhizal symbiosis efficiency of land plants accompanied the well-documented evolution of key morphological innovations [13] with a falling Palaeozoic [CO 2 ] a , as they transitioned from gametophyte- to sporophyte-dominant lifecycles. Our results, obtained with experiments on extant taxa ( Fig. 1 ), indicate that growth at 440 p.p.m. compared with 1,500 p.p.m. [CO 2 ] a penalized both species of basal non-vascular land plant lineage by reducing the efficiency of their AM symbiosis ( Fig. 5 ). At the same time, increasing sophistication in the form and function of vascular land plant shoots and roots enabled them to engage in a more efficient partnership with their obligate symbiotic fungal partners ( Fig. 5 ) to meet the rising host plant demand for P uptake. Quantification of AM efficiency for more species belonging to a broader suite of terrestrial plant lineages is required to better characterize how it changed, as Earth's floras and atmosphere evolved since the mid-Palaeozoic in partnership with symbiotic fungi to exploit soil phosphorus supplies. Nevertheless, our experimental evidence opens a new window on the consequences of plant–fungal evolution and [CO 2 ] a change for biogeochemical cycles in the past. It indicates that the co-evolution of root–fungal symbioses during the origin and diversification of embryophytes is likely to have progressively increased the efficiency of biogeochemical cycling of P in soil ecosystems. Plant species and growth conditions Preissia quadrata and Plantago lanceolata plants were collected from Anglesey dune slacks (Grid Reference SH 397 648). Marchantia paleacea plants were originally collected from cool temperate cloud forests, Vera Cruz, Mexico and mycorrhizal gemmae propagated from adults maintained in controlled environment growth chambers. Mature Osmunda regalis sporophytes were obtained from Burncoose Nursery, Cornwall. Plants of all species were cultivated in large pots (2 litres) filled with native Anglesey dune soil that acted as a natural mycorrhizal inoculum. Plastic cores of 20 mm diameter and 90 mm long with 10 μm pore size nylon mesh windows in their outer walls were filled with calcareous grassland soil and we installed a 1-mm diameter perforated-capillary tube centrally down each one. Four of these cores were inserted into each pot ( n =4 per species per [CO 2 ] a treatment) to surround the roots or rhizoids. A further mesh-core filled with glass wool was inserted into each pot to enable below-ground gas sampling throughout the 14 C labelling period. Each species was grown under [CO 2 ] a treatments of either 440 p.p.m. or 1,500 p.p.m. in controlled environment growth chambers (Conviron BDR16, Conviron, Canada). Each species was investigated with paired ambient and elevated [CO 2 ] a treatments. All plants were maintained with 18 °C/15 °C day/night temperatures and a 12-h day length. Both P. lanceolata and O. regalis were grown under an irradiance of 200 μmol m −2 s −1 , whereas P. quadrata and M. palaecea were grown at 50 μmol m −2 s −1 , which represent half light-saturating conditions for the vascular and non-vascular plant groups, respectively [39] , [40] . Plants were acclimated to growth chamber conditions for 12 weeks to allow mycorrhizal fungi networks to establish between roots/rhizoids and the mesh-walled soil cores. Molecular identification of fungal endosymbionts We extracted genomic DNA from thallus and root samples of stock and experimental plants using established methods [41] , with a purification step using GeneClean (QBioGene). We then amplified (PicoMaxx, Stratagene or JumpStart, Sigma), cloned (TOPO TA, Invitrogen) and sequenced (BigDye v.3 on ABI3730 Genetic Analyzer, Applied Biosystems) portions of fungal ribosomal RNA genes using nested-specific primer sets [42] and the fungal primers ITS1F [41] and ITS4 [43] (GLOMBS1670 5′-AGCTTTAACCGGCATCTGT-3′ ; ITS1F 5′-CTTGGTCATTTAGAGGAAGTAA-3′; ITS4 5′-TCCTCCGCTTATTGATATGC-3′; ITS4i 5′-TTGATATGCTTAAGTTCAGCG-3′; LETC1677 5′-CGGTGAGTAGCAATATTCG-3′; NS1 5′-GTAGTCATATGCTTGTCTC-3′; NS5 5′-AACTTAAAGGAATTGACGGAAG-3′; PARA1313 5′-CTAAATAGCCAGGCTGTTCTC-3′). We also screened and sequenced ca. 1600 bp of the fungal small ribosomal RNA gene using an approach described elsewhere [44] . Unique representative DNA sequences are deposited in GenBank Nucleotide Core database under accession numbers JQ811203 – JQ811206 . Phylogenetic analyses ( Figure 2 ) were conducted with PAUP version 4.0b10 (Phylogenetic Analysis Using Parsimony, Sinauer Associates, Massachusetts). Quantifying reciprocal plant 33 P for 14 C exchange Shoots were supplied with a pulse of 14 CO 2 for a 12-h photoperiod and 14 C tracked through the AM fungal network colonizing soil-filled mesh-walled cylinders that exclude rhizoids and roots. The reciprocal assimilation and transport of inorganic P from fungus-to-plant in the same soil compartments was quantified by supplying 33 P-orthophosphate into the mesh cores. In parallel control treatments, the cores were rotated to sever AM fungal network connections to the plants to account for diffusion of 14 C into, and 33 P out of, the cores. Standardized experimental design, [CO 2 ] a treatments, substrates and measurement protocols were rigorously employed to ensure direct comparability for all species. Following the acclimation period, we introduced 200 μl of 33 P-labelled orthophosphoric acid (1 MBq) into two of the soil-filled cores via the installed capillary tube to ensure even distribution of the isotope in each pot for ambient and elevated [CO 2 ] a -grown plant species. After 28 days, the soil cores were sealed with plastic caps and sterile anhydrous lanolin. The glass-wool-filled core was sealed using a gas-tight rubber septum (SubaSeal, Sigma) to allow non-destructive continuous monitoring by gas sampling of below-ground respiration. Each of the four replicate pots of mature plants for a particular [CO 2 ] a treatment was then sealed into a gas-tight labelling chamber and 1.1 MBq 14 C pulse label provided via liberation of 14 CO 2 from 15 μl Na 14 CO 3 using 2 ml lactic acid introduced to the chamber. Pots with mesh cores were maintained under growth chamber conditions and 1 ml of labelling chamber gas sampled through the septa to monitor 14 C drawdown after 1 h and every 4 h thereafter. One ml of gas from the glass wool-filled core in each pot was sampled after 1 h, and every 2 h thereafter to monitor below-ground respiration. Gas samples were injected into evacuated scintillation vials containing 10 ml Carbosorb (Perkin Elmer, Beaconsfield, UK) to trap CO 2 and then 10 ml Permafluor scintillation cocktail (Perkin Elmer) was added. Radioactivity was measured via liquid scintillation counting (Packard Tri-carb 3100TR, Isotech). Pots were left in situ until maximum 14 C flux was detected in the glass wool-filled core (between 12–14 h post-labelling), at which point cores were removed from the pots and incubated in airtight containers with 2 ml 2 M KOH to trap respired 14 C. Cores were transferred to fresh containers/KOH traps every 2 h for a further 6 h. From the KOH used to trap CO 2 , 1 ml was transferred to a scintillation vial with 10 ml Ultima Gold scintillation cocktail and the radioactivity monitored using liquid scintillation counting (Packard Tri-carb 3100TR, Isotech). Plant harvest and tissue analysis Upon removal of the soil cores from pots, all plant and soil material was separated into its constituent parts (that is, above-ground tissues, below-ground tissues, bulk soil), freeze dried and weighed. Homogenized freeze-dried sample (10–30 mg of plant tissue or soil) was digested in 1 ml concentrated sulphuric acid and heated to 365 °C for 15 min. On cooling 100 μl hydrogen peroxide was added to each sample and reheated at 365 °C to produce a clear solution, which was diluted up to 10 ml with distilled water. We mixed 2 ml of diluted digest with 10 ml of the liquid scintillant (Emulsify-safe, Perkin-Elmer) for quantification of 33 P activity (Packard Tri-carb 3100TR, Isotech). Precise 33 P content was quantified using the following formula [45] : where M 33 P=Mass of 33 P (mg), c DPM=counts as disintegrations per minute, S Act=specific activity of the source (Bq mmol −1 ), Df=dilution factor and Mwt=molecular mass of P. To quantify 14 C present within each component of the experimental pots, between 10 and 100 mg dry weight (dw) tissue was placed in Combusto-cones (Perkin Elmer) and the 14 C content measured through oxidation of each sample (Model 307 Packard Sample Oxidiser; Isotech). CO 2 released through oxidation was trapped in 10 ml Carbosorb (Perkin Elmer) before being mixed with 10 ml Permafluor (Perkin Elmer). Radioactivity present in the sample was measured through liquid scintillation counting (Packard Tri-carb 3100TR, Isotech). Total C fixed by the plant and transferred to the AM fungal network was calculated as a function of the total volume and CO 2 content of the labelling chamber and the proportion of the supplied 14 CO 2 label fixed by the plants. The difference in C between static cores and rotated cores is equivalent to the total C transferred from plant to symbiotic fungus within the soil core. The total amount of C ( 12 C and 14 C) assimilated by the plant and transferred to the fungus [46] was calculated using equations (2), (3) and (4): where T fp =total carbon transferred from fungus to plant (g); A =radioactivity of the tissue sample (Bq); A sp =specific activity of the source (Bq mol 1 ) and m a= atomic mass of 14 C (14). where P r =proportion of the total 14 C label supplied present in the tissue; m c =mass of C in the CO 2 present in the labelling chamber (g) (from the ideal gas law; equation (4)): where m cd =mass of CO 2 (g), M cd =molecular mass of CO 2 (44.01 g mol −1 ), P =pressure (kPa); V cd =volume of CO 2 in the chamber (0.003 m 3 ); m c =mass of unlabelled C in the labelling chamber (g); M , molar mass ( M of C=12.011 g); R =universal gas constant (J K −1 mol −1 ); T , absolute temperature (K); m c , mass of C in the CO 2 present in the labelling chamber (g), where 0.27292 is the proportion of C in CO 2 on a mass fraction basis, that is, 27.292%. Statistical analyses Differences between [CO 2 ] a treatments and species were calculated and analysed with two-way ANOVA using additional post-hoc Tukey testing where appropriate (for example, species×CO 2 interactions), in Minitab v12.21 (Minitab, US). Assumptions of normality and homogeneity of variances were met through log 10 transformations of variables where necessary. Accession codes: The sequencing data have been deposited in GenBank Nucleotide Core database under accession codes JQ811203 to JQ811206 . How to cite this article: Field, K.J. et al . Contrasting arbuscular mycorrhizal responses of vascular and non-vascular plants to a simulated Palaeozoic CO 2 decline. Nat. Commun. 3:835 doi: 10.1038/ncomms1831 (2012).